Induction of pluripotency in human somatic cells via a transient state resembling primitive streak-like mesendoderm During mammalian embryonic development, the primitive streak initiates the differentiation of pluripotent epiblast cells into germ layers. Pluripotency can be reacquired in committed somatic cells using a combination of a handful of transcription factors, such as OCT3/4, SOX2, KLF4 and c-MYC (hereafter referred to as OSKM), albeit with low efficiency. Here we show that during OSKM-induced reprogramming towards pluripotency in human cells, intermediate cells transiently show gene expression profiles resembling mesendoderm, which is a major component of the primitive streak. Based on these findings, we discover that forkhead box H1 (FOXH1), a transcription factor required for anterior primitive streak specification during early development, significantly enhances the reprogramming efficiency of human fibroblasts by promoting their maturation, including mesenchymal to epithelial transition and the activation of late pluripotency markers. These results demonstrate that during the reprogramming process, human somatic cells go through a transient state that resembles mesendoderm. Ectopic expression of transcription factors including OCT3/4, SOX2, KLF4 and c-MYC (hereafter referred to as OSKM) can invoke latent pluripotency of differentiated somatic cells albeit at low efficiency [1] , [2] . The inefficiency of reprogramming has suggested that elimination of epigenetic barriers and/or undefined secondary events are required in addition to OSKM [3] , [4] . However, the contamination by non-reprogrammed cells, which is major component of reprogramming cultures, impedes the understanding of molecular mechanisms of reprogramming, since non-reprogrammed cells exhibit different characteristics including gene expression and epigenetic statuses from bona fide iPSCs. Therefore, it has been difficult to observe the truly significant events occurring only in the reprogrammed cells. Recent works provided a concept of intermediate reprogrammed cell collection using specific cell surface antigens. Mouse intermediate reprogrammed cells can be labelled by stage-specific embryonic antigen (SSEA)-1 that is recognized as a specific marker of mouse embryonic stem cells (ESCs)/iPSCs [5] , [6] , [7] . We demonstrated that human cells positive (+) for tumor-related antigen (TRA)-1-60 [8] , [9] induced by OSKM are intermediate reprogrammed cells to being iPSCs [10] . Behaviour of TRA-1-60 (+) intermediate reprogrammed cells suggested that maturation, but not the initiation step, is a bottleneck of cell fate conversion towards human iPSCs. However, little is known about the characteristics of intermediate reprogrammed cells. In the current study, we purified TRA-1-60 (+) intermediate reprogrammed cells, which are candidates for bona fide iPSCs. Gene expression analyses revealed that mesendodermal genes are transiently activated during reprogramming, and re-suppressed in iPSCs. These findings led us discover that forkhead box H1 (FOXH1), a transcription factor that is essential for primitive streak specification, facilitates iPSC generation by promoting the maturation of intermediate reprogrammed cells including the mesenchymal to epithelial transition (MET) and the expression of marker genes for the late phase of reprogramming. These data demonstrate that the transient primitive streak-like mesendodermal (PSMN) state is crucial for the maturation of reprogrammed cells. The presence of large numbers of non-reprogrammed cells during the generation of iPSCs inhibits the accurate analysis of the reprogramming process. To overcome this issue, we used TRA-1-60 to capture cells being reprogrammed ( Fig. 1a ). Human dermal fibroblasts (HDFs) were transduced with OSKM retroviruses, transferred onto SNL feeder cells on day 7, and cultured under the conditions for ESCs thereafter. As part of our conventional protocol to generate iPSCs, we pick up colonies on around day 28 and continue cultivation for >20 passages to establish iPSC lines. In the current study, we analysed the proportion of TRA-1-60 (+) cells on various days by flow cytometry, and collected positive cells by using TRA-1-60 antibody-conjugated magnetic beads. A small population of TRA-1-60 (+) cells was detected on day 7, and then gradually increased in quantity and intensity ( Fig. 1b , Supplementary Fig. 1 ). The ability of TRA-1-60 (+) cells to form iPSC colonies also gradually increased and reached an efficiency similar to that of ESCs/iPSCs on day 20 or 28 ( Fig. 1c ). These results demonstrated that TRA-1-60 (+) cells were being reprogrammed toward iPSCs. 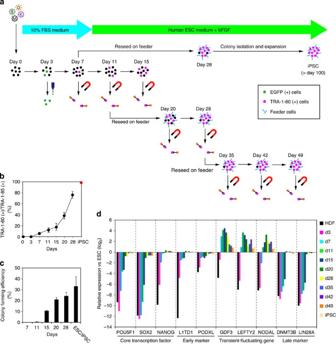Figure 1: TRA-1-60 (+) cells as an origin of human iPSCs. (a) A schematic drawing of TRA-1-60 (+) intermediate cells throughout human cellular reprogramming. (b) The proportion of TRA-1-60 (+) cells in human reprogramming cultures. Shown are the average proportions of TRA-1-60 (+) cells expressing TRA-1-85, which is a pan-human cell marker.N=3. (c) The efficiencies of iPSC generation from single TRA-1-60 (+) cells at each time point. The colony forming efficiencies were estimated by the number of iPSC colony-formed wells in single TRA-1-60 (+) cell sorted 96-well plates.N=3. (d) The expression of pluripotency-associated genes in TRA-1-60 (+) cells. The mean expressions from three microarray data sets for each time point, normalized to the levels of ESCs are shown. Figure 1: TRA-1-60 (+) cells as an origin of human iPSCs. ( a ) A schematic drawing of TRA-1-60 (+) intermediate cells throughout human cellular reprogramming. ( b ) The proportion of TRA-1-60 (+) cells in human reprogramming cultures. Shown are the average proportions of TRA-1-60 (+) cells expressing TRA-1-85, which is a pan-human cell marker. N =3. ( c ) The efficiencies of iPSC generation from single TRA-1-60 (+) cells at each time point. The colony forming efficiencies were estimated by the number of iPSC colony-formed wells in single TRA-1-60 (+) cell sorted 96-well plates. N =3. ( d ) The expression of pluripotency-associated genes in TRA-1-60 (+) cells. The mean expressions from three microarray data sets for each time point, normalized to the levels of ESCs are shown. Full size image In TRA-1-60 (+) cells, the expression of pluripotent stem cell markers, such as NANOG and endogenous OCT3/4 , progressively increased ( Fig. 1d and Supplementary Fig. 2 ). The transgene expression levels of the OSKM retroviruses peaked during day 7 and 15, and then became silenced by day 28 ( Supplementary Fig. 3 ). These data confirmed the gradual progression of reprogramming in TRA-1-60 (+) cells. Unexpectedly, however, we found that several pluripotent stem cell marker genes, such as GDF3 , LEFTY2 and NODAL , showed much higher expression levels in TRA-1-60 (+) cells than in iPSCs or ESCs ( Fig. 1d and Supplementary Fig. 2 ). This may suggest that TRA-1-60 (+) cells enter a transient state during reprogramming. To further explore this possibility, we compared the global gene expression profiles of TRA-1-60 (+) cells purified on various days, original HDFs, established iPSCs and differentiated progenies (endoderm, EN; mesoderm, ME; neuroectoderm, NE; and primitive streak-like mesendoderm [11] , [12] , [13] , [14] , PSMN from ESCs/iPSCs using DNA microarrays ( Supplementary Fig. 4 ). The principle component analysis (PCA) revealed that the expression levels of significant number of genes in TRA-1-60 (+) cells were not intermediate between HDFs and iPSCs, but were transiently activated or suppressed during iPSC generation (Component 1 in Fig. 2a ). The gene ontology analyses demonstrated that many of the transiently downregulated genes were related to metabolic processes ( Supplementary Fig. 5 ) [15] . On the other hand, many of the transiently activated genes were related to developmental processes ( Supplementary Fig. 5 ). 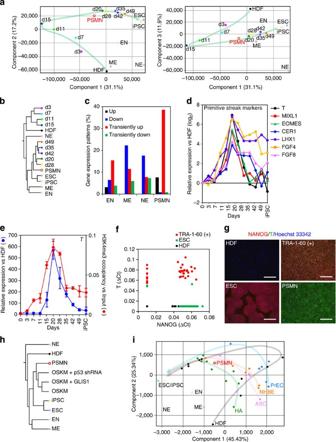Figure 2: The transient mesendodermal status of intermediate reprogrammed cells. (a) Comparison of the global gene expression between TRA-1-60 (+) cells and germ layers. Shown are PCA of the global gene expression in parental HDFs, TRA-1-60 (+) cells at the indicated time points, ESCs/iPSCs and differentiated cells, such as PSMN, EN, ME and NE. (b) Shown are the hierarchical clustering results of the global gene expression in parental HDFs, TRA-1-60 (+) cells at the indicated time points, ESCs/iPSCs and differentiated cells, such as PSMN, EN, ME and NE. (c) PSMN-enriched genes transiently upregulated in TRA-1-60 (+) cells. Shown are the percentages of ever-upregulated (black), ever-downregulated (blue), transiently upregulated (red) and transiently downregulated (green) genes in the enriched genes of PSMN, EN, ME or NE. (d) The expression of representative primitive streak marker genes during reprogramming. Shown are the relative expression levels of selected marker genes in TRA-1-60 (+) cells compared with parental HDFs. In these analyses, the averages of three microarray data set for each sample were used. (e) The expression and active histone marks ofTgene during reprogramming. Blue circles indicate the relative expression ofTcompared with that in HDFs. Red diamonds indicate the occupancy of H3K4me3 at the promoter region ofTgene.N=3. (f) The single-cell expression ofT. The expression ofNANOGandTin single HDFs and TRA-1-60 (+) cells on day 20 and ESCs. Each dot indicates one cell sample. The relative expression levels are shown as the ΔCt from qPCR. (g) Immunocytochemistry of T protein. The expression of NANOG (red) and T (green) in HDFs, TRA-1-60 (+) cells on day 20, ESCs and ESC-derived PSMN were analysed by immunocytochemistry. Nuclei were visualized by staining with Hoechst 33,342 (blue). Scale bars indicate 100 μm. (h) Booster-supported reprogramming via primitive streak-like state. The results of the hierarchical clustering analysis of the global gene expression in parental HDFs are shown, TRA-1-60 (+) cells on day 20 following transduction with OSKM, OSKM+GLIS1 and OSKM+p53 shRNA, ESCs/iPSCs and differentiated cells such as PSMN, EN, ME and NE. (i) The PCA of the microarray expression data from TRA-1-60 (+) cells at each time point, parental cell lines (HDF, HA, ASC, NHBE and PrEC), ESCs/iPSCs and differentiated cells such as PSMN, EN, ME and NE. Each arrow indicates the putative direction of the reprogramming progression. Figure 2: The transient mesendodermal status of intermediate reprogrammed cells. ( a ) Comparison of the global gene expression between TRA-1-60 (+) cells and germ layers. Shown are PCA of the global gene expression in parental HDFs, TRA-1-60 (+) cells at the indicated time points, ESCs/iPSCs and differentiated cells, such as PSMN, EN, ME and NE. ( b ) Shown are the hierarchical clustering results of the global gene expression in parental HDFs, TRA-1-60 (+) cells at the indicated time points, ESCs/iPSCs and differentiated cells, such as PSMN, EN, ME and NE. ( c ) PSMN-enriched genes transiently upregulated in TRA-1-60 (+) cells. Shown are the percentages of ever-upregulated (black), ever-downregulated (blue), transiently upregulated (red) and transiently downregulated (green) genes in the enriched genes of PSMN, EN, ME or NE. ( d ) The expression of representative primitive streak marker genes during reprogramming. Shown are the relative expression levels of selected marker genes in TRA-1-60 (+) cells compared with parental HDFs. In these analyses, the averages of three microarray data set for each sample were used. ( e ) The expression and active histone marks of T gene during reprogramming. Blue circles indicate the relative expression of T compared with that in HDFs. Red diamonds indicate the occupancy of H3K4me3 at the promoter region of T gene. N =3. ( f ) The single-cell expression of T . The expression of NANOG and T in single HDFs and TRA-1-60 (+) cells on day 20 and ESCs. Each dot indicates one cell sample. The relative expression levels are shown as the ΔCt from qPCR. ( g ) Immunocytochemistry of T protein. The expression of NANOG (red) and T (green) in HDFs, TRA-1-60 (+) cells on day 20, ESCs and ESC-derived PSMN were analysed by immunocytochemistry. Nuclei were visualized by staining with Hoechst 33,342 (blue). Scale bars indicate 100 μm. ( h ) Booster-supported reprogramming via primitive streak-like state. The results of the hierarchical clustering analysis of the global gene expression in parental HDFs are shown, TRA-1-60 (+) cells on day 20 following transduction with OSKM, OSKM+GLIS1 and OSKM+p53 shRNA, ESCs/iPSCs and differentiated cells such as PSMN, EN, ME and NE. ( i ) The PCA of the microarray expression data from TRA-1-60 (+) cells at each time point, parental cell lines (HDF, HA, ASC, NHBE and PrEC), ESCs/iPSCs and differentiated cells such as PSMN, EN, ME and NE. Each arrow indicates the putative direction of the reprogramming progression. Full size image The PCA and the hierarchical clustering demonstrated that that TRA-1-60 (+) cells on days 20–49 were most similar to mesendodermal cells derived from iPSCs, rather than undifferentiated iPSCs ( Fig. 2a,b ). The correlation coefficient of the global gene expression between TRA-1-60 (+) cells on day 20 and PSMN was 0.9718, which was comparable with clonal variations among ESC/iPSC lines (0.9634–0.9862) ( Supplementary Tables 1 and 2 ). In addition, we extended our comparison to 24 human fetal or adult tissues, and eight tissue-derived cells, in addition to the four ESC/iPSC-derived differentiated cells ( Supplementary Fig. 6 ). The highest similarity was observed between TRA-1-60 (+) cells (days 20–49) and PSMN. Approximately 40% of the PSMN-enriched genes were included in the transiently upregulated genes in TRA-1-60 (+) cells ( Fig. 2c ). We then checked the expression levels of marker genes for various developmental lineages. Marker genes for primitive streak, such as BRACHYURY ( T ) , MIXL1, CER1, LHX1 and EOMES showed a transient activation during iPSC generation in TRA-1-60 (+) cells ( Fig. 2d ). In contrast, marker genes for other lineages, including pluripotent stem cells, ME, EN and neuroectoderm, did not show such transient changes ( Supplementary Fig. 7 ). Quantitative reverse transcription polymerase chain reaction confirmed the transient activation of primitive streak-related genes in TRA-1-60 (+) cells ( Fig. 2e , Supplementary Fig. 8 ). The occupancy of trimethylated lysine 4 of histone H3 (H3K4me3), which is a mark of an activated promoter, transiently increased in primitive streak-related gene loci during reprogramming ( Fig. 2e , Supplementary Fig. 8 ). Single-cell quantitative reverse transcription polymerase chain reaction and immunocytochemistry revealed that virtually all of TRA-1-60 (+) cells on day 20, but not HDFs or ESCs, expressed T ( Fig. 2f,g ). These data suggest that TRA-1-60 (+) cells possess gene expression profiles resembling PSMN during the late stage of reprogramming. TRA-1-60 (+) cells induced by OSKM, along with GLIS1 or short hairpin RNA (shRNA)-mediated depletion of p53 (p53 shRNA), two of the strongest enhancers of reprogramming, were also clustered with PSMN ( Fig. 2h ) [16] , [17] , [18] , [19] , [20] , [21] . In addition, TRA-1-60 (+) cells derived from adipose-derived stem cells (ASC), as well as non-mesodermal lineages, such as astrocytes (HA, ectoderm), bronchial epithelium (NHBE, EN) and prostate epithelial cells (PrEC, EN), showed similarities to the PSMN in terms of the global gene expression ( Fig. 2i and Supplementary Fig. 9 ). Therefore, nascent human reprogrammed cells exhibit PSMN features, regardless of the reprogramming factors used or germ layer of original human somatic cells. The hierarchical clustering demonstrated that the TRA-1-60 (+) cells in early phases of reprogramming (days 3–15) resembled epithelial cells, including epidermis (EDM), PrEC and NHBE (green box in Supplementary Fig. 6 ). 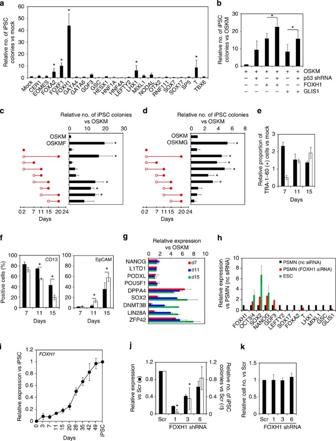Figure 3: Facilitation of the reprogramming efficiency by FOXH1. (a) FOXH1 facilitates iPSC generation. Shown are the relative numbers of iPSC colonies on day 24.N=3. *P<0.05 vs Mock (pairedt-test). (b) The action of FOXH1 is independent of that of p53. Shown are the relative numbers of iPSC colonies on day 24.N=3. *P<0.05 (pairedt-test). (c) FOXH1 enhances reprogramming in the late stage. We added 100 nM of dexamethasone (Dex) into the medium of HDFs transduced with OSKM and FOXH1GR from the time indicated by open circles until that indicated by closed circles. Shown are the relative numbers of iPSC colonies on day 24.N=3. *P<0.05 vs OSKM (pairedt-test). (d) GLIS1 enhances reprogramming in the early stage. We performed same kind of experiments toFigure 3cusing GLIS1GR instead of FOXH1GR.N=3. *P<0.05 vs OSKM (pairedt-test). (e) FOXH1 increases TRA-1-60 (+) cells in the late stage. Shown are the relative proportions of TRA-1-60 (+) cells induced by OSKMG (closed bars) or OSKMF (opened bars).N=3. (f) FOXH1 promotes the epithelialization during reprogramming. Shown are the proportions of CD13 (+) or EpCAM (+) cells in the TRA-1-60 (+) cell population carrying OSKM (closed bars) or OSKMF (open bars) by flow cytometry.N=3. *P<0.05 (pairedt-test). (g) FOXH1 enhances the expression of late reprogramming markers. Shown are the relative expression levels in TRA-1-60 (+) cells induced by OSKMF normalized toG3PDHexpression.N=3. (h) FOXH1 is required for PSMN differentiation. Shown are the relative expression levels in PSMN differentiated from FOXH1 small interfering RNA-transduced ESCs/iPSCs normalized toG3PDHexpression.N=3. (i) The expression of endogenous FOXH1 in TRA-1-60 (+) cells. Shown are the relative expression levels of FOXH1 normalized toG3PDHexpression.N=3. (j) Endogenous FOXH1 is required for iPSC generation. We introduced OSKM, along with scramble shRNA (Scr) or FOXH1 shRNAs (1, 3 or 6), into HDFs. On day 15, the knockdown efficiencies were evaluated by qRT–PCR (closed bars). Each value was normalized to that ofG3PDH. The open bars indicate the relative numbers of iPSC colonies on day 24.N=3. *P<0.05 versus Scr (pairedt-test). (k) FOXH1 does not affect HDF proliferation. Shown are the relative numbers of HDFs transduced with OSKM in combination with pMKO.1-puro encoding scramble shRNA (Scr) and FOXH1 shRNA1, 3 or 6 on day 7. Each value was normalized to that ofG3PDH.N=3. The correlation coefficient between TRA-1-60 (+) cells on days 3–15 and EDM, PrEC and NHBE were 0.9082–0.9105, 0.8989–0.9052 and 0.9033–0.9106, respectively ( Supplementary Table 3 ). We also observed suppression of mesenchymal genes and activation of epithelial genes during this period [22] , [23] ( Supplementary Fig. 10 ). Taken together, these data suggest that epithelialization is one of the dominant events that occur in TRA-1-60 (+) intermediate cells during the early phases of reprogramming. This result may explain a recent report arguing that there was a transient EDM-like status during mouse cell reprogramming [6] . Our findings led us to hypothesize that transcription factors that play important roles in mesendoderm and primitive streak may facilitate iPSC generation. We selected 23 transcription factors that were highly expressed in mesendoderm and transduced each one of them, together with OSKM, into HDFs ( Fig. 3a ). We found that five factors, including FOXA2, FOXF1, FOXH1, LHX1 and T, significantly increased the numbers of iPSC colonies. Among them, FOXH1 showed the strongest effect. FOXH1 functions as a downstream target of the Nodal signal and is required for the specification of anterior primitive streak [24] , [25] . The effect of FOXH1 in increasing iPSC colonies was comparable with those of p53 shRNA and GLIS1 ( Fig. 3b and Supplementary Fig. 11 ) [16] , [17] , [18] , [19] , [20] , [21] . Figure 3: Facilitation of the reprogramming efficiency by FOXH1. ( a ) FOXH1 facilitates iPSC generation. Shown are the relative numbers of iPSC colonies on day 24. N =3. * P <0.05 vs Mock (paired t -test). ( b ) The action of FOXH1 is independent of that of p53. Shown are the relative numbers of iPSC colonies on day 24. N =3. * P <0.05 (paired t -test). ( c ) FOXH1 enhances reprogramming in the late stage. We added 100 nM of dexamethasone (Dex) into the medium of HDFs transduced with OSKM and FOXH1GR from the time indicated by open circles until that indicated by closed circles. Shown are the relative numbers of iPSC colonies on day 24. N =3. * P <0.05 vs OSKM (paired t -test). ( d ) GLIS1 enhances reprogramming in the early stage. We performed same kind of experiments to Figure 3c using GLIS1GR instead of FOXH1GR. N =3. * P <0.05 vs OSKM (paired t -test). ( e ) FOXH1 increases TRA-1-60 (+) cells in the late stage. Shown are the relative proportions of TRA-1-60 (+) cells induced by OSKMG (closed bars) or OSKMF (opened bars). N =3. ( f ) FOXH1 promotes the epithelialization during reprogramming. Shown are the proportions of CD13 (+) or EpCAM (+) cells in the TRA-1-60 (+) cell population carrying OSKM (closed bars) or OSKMF (open bars) by flow cytometry. N =3. * P <0.05 (paired t -test). ( g ) FOXH1 enhances the expression of late reprogramming markers. Shown are the relative expression levels in TRA-1-60 (+) cells induced by OSKMF normalized to G3PDH expression. N =3. ( h ) FOXH1 is required for PSMN differentiation. Shown are the relative expression levels in PSMN differentiated from FOXH1 small interfering RNA-transduced ESCs/iPSCs normalized to G3PDH expression. N =3. ( i ) The expression of endogenous FOXH1 in TRA-1-60 (+) cells. Shown are the relative expression levels of FOXH1 normalized to G3PDH expression. N =3. ( j ) Endogenous FOXH1 is required for iPSC generation. We introduced OSKM, along with scramble shRNA (Scr) or FOXH1 shRNAs (1, 3 or 6), into HDFs. On day 15, the knockdown efficiencies were evaluated by qRT–PCR (closed bars). Each value was normalized to that of G3PDH . The open bars indicate the relative numbers of iPSC colonies on day 24. N =3. * P <0.05 versus Scr (paired t -test). ( k ) FOXH1 does not affect HDF proliferation. Shown are the relative numbers of HDFs transduced with OSKM in combination with pMKO.1-puro encoding scramble shRNA (Scr) and FOXH1 shRNA1, 3 or 6 on day 7. Each value was normalized to that of G3PDH . N =3. Full size image We previously reported that mouse Glis1 was specifically expressed in unfertilized oocytes in mice, and that it facilitated iPSC generation through promoting the expression of pluripotency-associated genes [26] . In this study, we found that GLIS1 was highly expressed in PSMN derived from human ESCs/iPSCs ( Supplementary Fig. 12a ). We also found that mouse Glis1 is expressed in embryonic regions, including primitive streak ( Supplementary Fig. 12b ). Forced expression of GLIS1 in human ESCs gave rise to PSMN features ( Supplementary Fig. 12c,d,e ). These data demonstrated that GLIS1 has important roles in the PSMN lineage, which may contribute to its pro-reprogramming activity. In addition, the stage-specific activation of FOXH1 demonstrated that FOXH1 clearly facilitated the reprogramming efficiency in late stages ( Fig. 3c ). These results are in contrast to those using GLIS1, which facilitated reprogramming in the earlier stages and increased the proportion of TRA-1-60 (+) cells ( Fig. 3d,e ). This may suggest that GLIS1 promotes the induction of a primitive streak-like state, whereas FOXH1 promotes the maturation of cells in this state. In fact, the proportion of TRA-1-60 (+) cells was reproducibly reduced by FOXH1 on day 7, but the proportion was increased again on days 11 and 15 compared with cells transduced with OSKM alone ( Fig. 3e ). We found that FOXH1 promoted the downregulation of a fibroblast marker, CD13, and the upregulation of an epithelial marker, EpCAM, in TRA-1-60 (+) cells on days 11 and 15 ( Fig. 3f ). In addition, the expression of late reprogramming markers, such as DPPA4 , DNMT3B , LIN28A , ZFP42 and endogenous SOX2 (ref. 7 ), were significantly enhanced by FOXH1 ( Fig. 3g ). These data further suggest that FOXH1 may enhance the reprogramming efficiency by facilitating the maturation of TRA-1-60 (+) cells. Next, we examined whether endogenous FOXH1 is required for human iPSC generation and PSMN differentiation. Knockdown of FOXH1 in ESCs significantly interfered with their differentiation into PSMN ( Fig. 3h ). The expression of endogenous FOXH1 was continuously increased in TRA-1-60 (+) cells during their reprogramming towards iPSCs ( Fig. 3i ). Three out of six shRNAs (1, 3 and 6) suppressed the expression of endogenous FOXH1 in ESCs or OSKM-transduced HDFs with ~90%, 70% and 50% efficiencies, respectively ( Fig. 3i and Supplementary Fig. 13 ). When co-introduced with OSKM, shRNA1 nearly abolished the generation of iPSC colonies ( Fig. 3j ). In addition, shRNA 3 decreased iPSC colony formation by 50%. In contrast, the suppression of FOXH1 did not ameliorate the proliferation of transduced HDFs ( Fig. 3k ). These data suggest that FOXH1 plays an important role in the reprogramming process towards iPSCs. We then examined the effects of other FOX family transcription factors on human iPSC generation. We found that five factors, including FOXA2, FOXB1, FOXF1, FOXG1 and FOXH1, out of 36 selected FOX genes significantly increased the numbers of iPSC colonies ( Supplementary Fig. 14 ). Similar to SOX, KLF and MYC families [27] , some of FOX family transcription factors have overlapping effects on human iPSC generation ( Supplementary Fig. 15 ). The use of FOXH1 along with OSKM for reprogramming did not alter the characteristics of the resulting iPSCs ( Supplementary Fig. 16 ). We examined whether mouse reprogramming also goes through a transient state. We reprogrammed mouse embryonic fibroblasts (MEFs) derived from Nanog-GFP transgenic mice [28] , and isolated nascent reprogrammed cells as SSEA-1 (+) and/or Nanog-GFP (+). The PCA and hierarchical clustering of the microarray data identified a component that indicates a transient change resembling PSMN during mouse iPSC generation ( Supplementary Fig. 17 ). In addition, by using a secondary iPSC induction system in mice, Polo et al. [5] reported that there was a transient activation of several genes, including T , Eomes and Mixl1 . In summary, our cell capture strategy for human intermediate reprogrammed cells revealed that they go through a transient state that resembles PSMN. During the maturation step, virtually all TRA-1-60 (+) cells expressed early mesendodermal genes. Such PSMN features gradually drained in further progression of reprogramming towards iPSC. Previous and our current study clearly show that the human reprogramming process takes more time than we thought it would and the maturation step is important [29] . Although we have little evidence for the inevitability of the transition, this observation led us to find FOXH1 as an enhancer of reprogramming. FOXH1 promoted the MET of TRA-1-60 (+) cells and the activation of late pluripotent markers. The epithelial to mesenchymal transition, which is an opposite phenomenon of MET, is a key event for differentiation of epiblasts into mesendoderm at primitive streak in embryonic development. FOXH1 may facilitate the reprogramming by promoting the reversion of somatic cell fate to PSMN state. Further understanding of the reprogramming process will enable more robust generation of human iPSCs. Statistical analyses We evaluated the data by paired t -tests using the Kaleidagraph software programme (HULINKS), and values of P <0.05 were considered to be significant (indicated by asterisks in figures). The error bars represent the standard deviation (s.d.). Cell culture We obtained HDFs from the Japanese Collection of Research Bioresources. HDFs, PLAT-E [30] , PLAT-GP and MEFs were maintained in Dulbecco’s modified Eagle medium (DMEM, Nacalai Tesque) containing 10% fetal bovine serum (FBS, Japan Bio Serum) and 0.5% penicillin and streptomycin (Pen/Strep, Life Technologies). ESC clones obtained from WiCELL [31] and Kyoto University [32] were maintained in Primate ESC medium (ReproCELL) supplemented with 4 ng ml −1 recombinant human basic fibroblast growth factor (bFGF, Wako) on mitomycin C (MMC)-inactivated SNL feeders [33] , or in mTeSR1 (Veritas) on Matrigel-coated plates (growth factor reduced, BD biosciences) as described previously [2] . Human epidermal keratinocytes (EDM, Lonza), astrocytes (HA, Cell applications), normal human bronchial epithelial cells (NHBE, Lonza), adipose tissue-derived stem cells (ASC, Life Technologies) and prostate epithelial cells (PrEC, Lonza) were maintained under the manufacturer’s recommended conditions. Mouse ESCs (1B4) and iPSCs (20D17) [28] were maintained in mESC medium consisting of 80% knockout DMEM (Life Technologies), 15% knockout serum replacement (KSR, Life Technologies), 1% Glutamax, 1% NEAA, 100 nM 2-ME, 0.5% Pen/Strep and 1,000 units ml −1 recombinant mouse leukaemia inhibitory factor (Millipore) on gelatinized plates. Reprogramming To generate retroviral particles, we introduced retroviral vectors into PLAT-E or PLAT-GP cells by using the FuGENE 6 transfection reagent (Roche) as per the manufacturer’s protocol. On the following day, the medium was replaced with fresh one and cells were incubated for another 24 h. The virus-containing supernatant was collected, filtered through a 0.45 μm pore size cellulose acetate filter (Whatman) and was supplemented with 4 μg ml −1 Polybrene (Nacalai Tesque). Then, we mixed appropriate combinations of viruses and used them to expose HDFs carrying the mouse Solute carrier family 7 (cationic amino-acid transporter, y+ system) member 1 ( Slc7a1 ) gene overnight. This point was designated as day 0. For the transduction of retroviruses into cell lines other than HDFs, we performed spinfection at 700 g for 1 h with the fusiogenic envelope G glycoprotein of the vesicular stomatitis virus (VSV-G)-pseudotyped pantropic viruses produced by PLAT-GP cells. To collect the samples on day 3 post transduction, we introduced pMXs-IRES-EGFP (IG) encoding SOX2 instead of pMXs-SOX2, along with OKM, and sorted EGFP (+) cells by flow cytometry. We harvested the cells on day 7 post transduction, and re-plated them onto MMC-inactivated SNL feeders to generate iPSCs. The following day, the medium was replaced with Primate ESC medium supplemented with 4 ng ml −1 bFGF, and the medium was changed every other day. To collect TRA-1-60 (+) cells, we performed magnetic-activated cell sorting with a TRA-1-60 antibody at each indicated time point. The number of iPSC colonies was counted on day 24 post transduction. We distinguished bona fide iPSC colonies from non-iPSC colonies by their morphological differences [2] , [17] , [26] , [27] , [34] , [35] . MEFs carrying Nanog-GFP [28] were introduced with OCT3/4, SOX2, KLF4, c-MYC and GLIS1 by retroviral transduction. Two days after infection, the medium was replaced with the mESC medium. We collected each fraction by using a SSEA-1 antibody and/or Nanog-GFP on the indicated days by flow cytometry [26] . The cells were passaged on days 7, 11, 15 and 20 at 1 × 10 6 cells per 100 mm dish. PSMN differentiation The differentiation of human ESCs/iPSCs into PSMN was performed as described previously [13] . In brief, single-cell suspensions of human ESCs/iPSCs were plated onto fibronectin-coated plates (BD biosciences) in DMEM/F12 supplemented with 1% Insulin–Transferrin–Selenite (ITS, Life Technologies), 1% Glutamax, 1% NEAA, 2% B27 (Life Technologies), 100 nM 2-ME and 0.5% Pen/Strep. We added 3 μM CHIR99021 (Stemgent) and 50 ng ml −1 Activin A (Peprotech) on day 1, 3 μM CHIR99021, 25 ng ml −1 Activin A and 20 ng ml −1 bFGF on day 2 and 3 μM, CHIR99021, 10 ng ml −1 Activin A, 20 ng ml −1 bFGF and 40 ng ml −1 BMP4 (R&D systems) on day 3. EN differentiation EN differentiation was performed as described previously, with slight modification [36] . The single-cell suspensions of human pluripotent stem cells were plated onto Matrigel-coated plates in RPMI1640 (Life Technologies) containing 2% B27, 100 ng ml −1 Activin A, 3 μM CHIR99021 and 0.5% Pen/Strep. We added 0.5 mM sodium butyrate (Sigma) on days 1–3, and then carried out sodium butyrate-free culture until day 7. ME differentiation ME differentiation was performed as described previously, with slight modification [37] . The single-cell suspensions of human pluripotent stem cells were plated onto Collagen I-coated plates (BD biosciences) in DMEM/F12 containing 2% B27, 100 ng ml −1 Activin A, 3 μM CHIR99021 and 0.5% Pen/Strep. Forty-eight hours later, the medium was replaced with DMEM/F12 supplemented with 2% B27, 25 ng ml −1 BMP4 and 0.5% Pen/Strep. The medium was changed every other day until day 8. NE differentiation NE differentiation protocol with dual SMAD inhibition was used according to previous reports [38] , [39] . The single-cell suspensions of pluripotent stem cells were transferred to Lipidure-coated low-binding 96-well plates (NOF corporation) in DMEM/F12 containing 5% KSR, 1% NEAA, 1% Glutamax, 100 nM 2-ME, 2 μM Dorsomorphin (Stemgent) and 10 μM SB431542 (Stemgent). The medium was changed on days 5, 8 and 11. The total differentiation period was 14 days. Flow cytometry and fluorescence-activated cell sorting We harvested the cells at the indicated time points by treatment with 0.25% trypsin/1 mM EDTA (Life Technologies) or Accutase (Life Technologies). Fixation and permeabilization were performed before antibody staining with 4% paraformaldehyde and 0.2% Triton X-100, respectively. At least 5 × 10 4 cells were analysed for quantification in all experiments using the FACS Aria II instrument (BD biosciences). Cell sorting was also performed using the FACS Aria II. We used the following antibodies for the studies: Alexa 488-conjugated TRA-1-60 (1:20, 560173, BD biosciences), Alexa 488-conjugated SSEA-4 (1:20, 506348, BD biosciences), fluorescein isothiocyanate (FITC)-conjugated TRA-2-49/6E (1:5, FCMAB133, Millipore), allophycocyanin (APC)-labelled TRA-1-85 (1:5, FAB3195A, R&D systems), APC-labelled anti-C-X-C chemokine receptor type 4 (CXCR4) antibody (1:5, FAB170A, R&D systems), PE-labelled anti-platelet-derived growth factor receptor alpha (PDGFRA) antibody (1:5, 556002, BD Pharmingen), APC-conjugated anti-BRACHYURY antibody (1:5, IC20851A, R&D systems), anti-polysialylated neuronal cell adhesion molecule (PSA-NCAM) antibody (1:50, MAB5324, Millipore), PE-conjugated CD13 antibody (1:5, 555394, BD biosciences), FITC-labelled CD326 (EpCAM) antibody (1:10, 130-080-301, Miltenyi biotec), PE-labelled SSEA-1 (560866, BD Pharmingen) and Alexa 647-conjugated anti-mouse IgM antibody (1:500, A-21238, Life Technologies). Magnetic-activated cell sorting The cells harvested by trypsinization were passed through a 40 μm pore size cell strainer (BD biosciences) to remove the cell debris. The cells were incubated with PE-conjugated TRA-1-60 (1:5, 560193, BD Pharmingen), and then with anti-PE microbeads (130-048-801, Miltenyi biotec). Cell separation was performed with the serial two column mode of an AutoMACS Pro system (Miltenyi biotec). After separation, we confirmed the purity by flow cytometry. Microarray and bioinformatics The total RNA was purified as described above, and then was evaluated using a 2100 Bioanalyzer (Agilent Technologies). Human tissue RNA panels were obtained from Clontech Laboratories. Fifty nanograms of total RNA was labelled with Cyanine 3-CTP and used for hybridization with SurePrint G3 Human GE 8 × 60 K (G4851A, Agilent Technologies) and Mouse GE 8 × 60 K (G4852A, Agilent Technologies) with the one colour protocol. The arrays were scanned with a Microarray Scanner System (G2565BA, Agilent Technologies), and extracted signals were analysed using the GeneSpring version 12.6 software programme (Agilent Technologies). Gene expression values were normalized by the 75th percentile shifts. The hierarchical clustering analyses were performed with a Euclidean distance and complete linkage clustering method. Differentially expressed genes in each lineage were extracted by comparison with the profiles in HDFs, ESCs and iPSCs by unpaired a t -tests with Benjamini and Hochberg corrections (significance set at P <0.05, fold change>2.0). Transiently activated or suppressed genes were narrowed down by cutting off the absolute rate of contribution in component 1 for values higher than 0.6. The gene ontology analyses were performed using the EASE programme on the DAVID bioinformatics database website ( http://www.david.abcc.ncifcrf.gov/home.jsp ). The multiple protein sequence alignment was performed using the CLUSTALW programme ( http://www.genome.jp/tools/clustalw/ ). Gene silencing For short-term gene silencing, Stealth small interfering RNA for FOXH1 (equal mixture of HSS189664, HSS113216 and HSS113217) or Negative control Mid GC (Life Technologies) was transfected into human ESCs/iPSCs using Lipofectamine RNAi Max (Life Technologies) according to the manufacturer’s protocol on day 0 of PSMN differentiation protocol. For stable knockdown during reprogramming, we introduced a pMKO.1-puro retroviral vector (#8452, Addgene) encoding shRNA against genes of interest, at the same time as the OSKM transduction. The sequences of FOXH1 shRNA 1, 3 and 6 were 5′-CACCTCCTACTTGCCTATCTA-3′, 5′-GCCTATCTACACTCCCAATGT-3′ and 5′-TGCAGCCTGTGAGGCTCTTAA-3′, respectively. Plasmid construction The open reading frames of the genes used in this study were amplified by PCR, subcloned into pENTR-D-TOPO (Life Technologies) and verified by sequencing. The open reading frames were transferred to expression vectors such as pMXs-gw or pMXs-gw-IP by using the Gateway LR reaction system (Life Technologies) according to the manufacturer’s protocol. To generate cGR-fused constructs, stop codon-lacking GLIS1 and FOXH1 were amplified by PCR and cloned into pCR2.1-TOPO (Life Technologies). An Eco RI/ Spe I fragment of each gene cloned in pCR2.1 and a Spe I/ Not I fragment of pPyCAG-cGR-IP were inserted into the Eco RI/ Not I site of pMXs. A knockdown vector for human p53 gene [40] (pMKO.1-puro p53 shRNA2, #10672) was purchased from Addgene. Quantitative reverse transcription polymerase chain reaction Total RNA was purified from cell lysates treated with the Qiazol reagent (Qiagen) by using a miRNeasy mini kit (Qiagen), and was incubated with the Turbo DNA free kit (Life Technologies) to remove genomic DNA. The reverse transcription reaction was performed with 1 μg of DNase-treated RNA using the ReverTra Ace-α kit (Toyobo) and oligo dT 20 primer. PCR was performed using SYBR premix Ex-Taq II (Takara) and a StepOne instrument (Applied Biosciences). The primer sequences for each gene are provided in Supplementary Table 4 . Embryoid body formation Small clumps of human ESCs/iPSCs were transferred to low-binding plates (Nunc) in DMEM/F12 (Life Technologies) containing 20% KSR, 1% Glutamax, 1% NEAA, 100 nM 2-ME and 0.5% Pen/Strep. The medium was changed every other day. After 8 days of floating culture, aggregates were transferred onto gelatinized plates and cultured for another eight days. The medium was changed every other day. Western blotting analyses Cell lysates were prepared using RIPA buffer (50 mM Tris–HCl, pH 8.0, 150 mM NaCl, 1% nonidet P-40, 1% sodium deoxycholate, and 0.1% SDS), supplemented with protease inhibitor cocktail (Roche). Thirty micrograms of denatured cell lysates were separated by electrophoresis on 12 or 14% SDS–polyacrylamide gels, and were transferred to polyvinylidene fluoride membranes (Millipore). The blot was blocked with TBST (20 mM Tris–HCl, pH 7.6, 136 mM NaCl, and 0.1% Tween-20) containing 1% skim milk and then incubated with primary antibody solution at 4 °C overnight. After washing with TBST, the membrane was incubated with horseradish peroxidase (HRP)-conjugated secondary antibody for 45 min at room temperature with constant agitation. Signals were raised with Immobilon Western HRP substrate (Millipore) and detected using a LAS3000 mini imaging system (FUJIFILM). Primary antibodies for p53 (1:200, sc-126, Santa Cruz), p21 (1:500, sc-397, Santacruz) and β-ACTIN (1:5,000, A5441, Sigma), and horseradish peroxidase-linked secondary antibodies for mouse immunoglobulin G (IgG) (1:3,000, #7076, Cell signalling technology) and rabbit IgG (1:2,000, #7074, Cell signalling technology) were used. Immunocytochemistry The cells were fixed with 4% paraformaldehyde and permeabilized with phosphate-buffered saline (PBS) containing 5% goat or donkey normal serum (Chemicon), 1% bovine serum albumin (BSA; Nacalai Tesque) and 0.2% Triton X-100 (Nacalai Tesque). Samples were incubated with primary antibodies against NANOG (1:100, RCAB003P, ReproCELL), T (1:100, AF2085, R&D systems) SOX17 (1:200, AF1924, R&D systems), α-smooth muscle actin (1:600, M085101, DAKO) and NESTIN (1:1,000, ab5968, Abcam), which were diluted in staining solution (PBS containing 1% BSA) at 4 °C overnight. After being washed with PBS, the samples were exposed to staining solution containing fluorescence-conjugated secondary antibodies such as Alexa 488-conjugated anti-goat IgG (1:500, A-11055, Life Technologies), Alexa 546-conjugated anti-mouse IgG (1:500, A-11030, Life Technologies), Alexa 488-conjugated anti-rabbit IgG (1:500, A-11034, Life Technologies) and Alexa 546-conjugated anti-rabbit IgG (1:500, A-11035, Life Technologies), as well as Hoechst 33342 (1 μg ml −1 , H3570, Life Technologies). Images were obtained using a BZ9000 imaging system (KEYENCE). Pyrosequencing Five hundred nanograms of purified genomic DNA was used for the bisulphite CT conversion with the EZ DNA methylation kit (Zymo Research) according to the manufacturer’s recommendations. The resultant DNA samples were used for PCR with biotinylated primers as templates, and amplified products were analysed by the Pyromark system (Qiagen). The primer sequences are provided in Supplementary Table 4 . Chromatin immunoprecipitation Approximately 3 × 10 5 cells were fixed with 1% formaldehyde and quenched with 125 mM glycine. Fixed cells were sequentially treated with LB1 (50 mM Hepes-KOH, pH 7.5, 140 mM NaCl, 1 mM EDTA, 10% glycerol, 0.5% Nonidet P-40 and 0.25% Triton X-100), LB2 (10 mM Tris–HCl, pH 8.0, 200 mM NaCl, 1 mM EDTA and 0.5 mM EGTA), LB3 (10 mM Tris–HCl, pH 8.0, 100 mM NaCl, 1 mM EDTA, 0.5 mM EGTA and 0.1% sodium deoxycholate) to obtain nuclear extracts. Chromatin samples were sheared by treatment with a Misonix Astrason S-3000 sonicator (On, 30 s; Off, 1 min; Power, 7.0; 15 cycles). We added 1/10 volume of 10% Triton X-100 solution to the cell lysates and obtained cleared supernatants after centrifugation. To reduce the non-specific background, we incubated the chromatin samples with normal mouse IgG (sc-2025, Santa Cruz) linked with Dynabeads M-280 Sheep Anti-Mouse IgG (102-01D, Life Technologies) for 30 min at 4 °C. After removal of the beads, the cleared lysates were incubated with a Dynabeads-conjugated anti-trimethylated lysine 4 of histone H3 antibody (MABI0304, Wako) overnight at 4 °C with constant rotation. After incubation, the beads were washed twice each with wash buffer 1 (20 mM Tris–HCl, 8.0, 150 mM NaCl, 2 mM EDTA, 1% TritonX-100 and 0.1% SDS), wash buffer 2 (20 mM Tris–HCl, pH 8.0, 500 mM NaCl, 2 mM EDTA, 1% Triton X-100 and 0.1% SDS), wash buffer 3 (10 mM Tris–HCl, pH 8.0, 250 mM lithium chloride, 1 mM EDTA, 1% Nonidet-P 40 and 1% sodium deoxycholate) and TE buffer (10 mM Tris–HCl, pH 8.0 and 1 mM EDTA). Then, we incubated the beads with elution buffer (25 mM Tris–HCl, pH 7.5, 5 mM EDTA and 0.5% SDS) supplemented with 0.4 mg ml −1 protease K (Nacalai Tesque) at 42 °C for 1 h, and then at 65 °C overnight with constant rotation. Eluates were purified using the Qiaquick PCR purification kit (Qiagen) and were used for PCR as templates. The primer sequences are provided in Supplementary Table 4 . Teratoma formation and histological analyses Approximately 3 × 10 5 harvested cells suspended in DMEM/F12 containing 10 μM Y-27632 (Wako) were injected into the testes of severe combined immunodeficient male mice (6 weeks old) by using a Hamilton syringe [41] . Animal experiments were approved by Kyoto University ethical committee (Approved number is K3-12). After 8–10 weeks, the tumours were dissected and fixed with 4% paraformaldehyde and 70% ethanol in sequence. Paraffin-embedded sections were stained with hematoxylin and eosin. Images were obtained by using a BZ9000 system. Single-cell manipulation Single-cell suspensions prepared by trypsinization were incubated with PE-conjugated TRA-1-60 and 4′,6-diamidino-2-phenylindole (Life Technologies). TRA-1-60 (+)/4′,6-diamidino-2-phenylindole (−) cells were directly sorted onto MMC-treated SNL feeders in human ESC medium supplemented with 4 ng ml −1 bFGF and 10 μM Y-27632 for the colony formation assay, or into PCR master mix for the single-cell expression analyses using the FACS Aria II instrument. The template for the single-cell PCR was prepared using the Cellsdirect Reagent (Life Technologies) according to the manufacturer’s protocol. Pre-amplification of the target sequences was performed for 22 cycles. The subsequent PCR and data collection were conducted with a Biomark system (Fluidgm). Each sample was validated based on the expression of either G3PDH or ACTB, with Ct value less than 15. The Ct values higher than 26 were considered to indicate no expression and were unified as 100 for the calculation of the ΔCt. The Taqman assays used in this study are shown in Supplementary Table 5 . Accession codes : The microarray data have been deposited in Gene Expression Omnibus under accession number GSE50206 . How to cite this article: Takahashi, K. et al. Induction of pluripotency in human somatic cells via a transient state resembling primitive streak-like mesendoderm. Nat. Commun. 5:3678 doi: 10.1038/ncomms4678 (2014).